Engineering modular and orthogonal genetic logic gates for robust digital-like synthetic biology Modular and orthogonal genetic logic gates are essential for building robust biologically based digital devices to customize cell signalling in synthetic biology. Here we constructed an orthogonal AND gate in Escherichia coli using a novel hetero-regulation module from Pseudomonas syringae . The device comprises two co-activating genes hrpR and hrpS controlled by separate promoter inputs, and a σ 54 -dependent hrpL promoter driving the output. The hrpL promoter is activated only when both genes are expressed, generating digital-like AND integration behaviour. The AND gate is demonstrated to be modular by applying new regulated promoters to the inputs, and connecting the output to a NOT gate module to produce a combinatorial NAND gate. The circuits were assembled using a parts-based engineering approach of quantitative characterization, modelling, followed by construction and testing. The results show that new genetic logic devices can be engineered predictably from novel native orthogonal biological control elements using quantitatively in-context characterized parts. As Boolean logic gates are widely used in electronic circuits to build digital devices, logic operations are encoded in gene regulatory networks that cells use to cascade and integrate multiple environmental and cellular signals [1] , [2] , [3] and to respond accordingly. Thus, by designing customized genetic logic circuits to link various cellular sensors and actuators, we can program living cells to generate precise desired behaviours in response to specific extra or intra-cellular signalling inputs [2] , [4] . In particular, multiple-input genetic logic gates are necessary for cells to recognize complex conditions that are normally specified by a combination of several signals (for example, pH, temperature, small molecules or metal ions), and thus can greatly improve the sensing specificity and increase the accuracy of biological control. For example, various environmental pollutant-like arsenic [5] , xylene [6] and Pseudomonas aeruginosa -responsive [7] sensors can be wired to a multiple-input AND gate, allowing cells to report and neutralize a combinatorial toxic circumstance. The AND gate inputs can also be connected to certain disease-related signal responsive promoters [8] and the output to a therapeutic gene to achieve highly specific in vivo targeting [9] and curing of diseased cells. Furthermore, multiple logic gates can be combined to build larger information-processing circuits with advanced cellular functions, such as a projected image edge detector [10] and even a cellular event counter. To date, a number of synthetic gene circuits [11] , [12] , [13] , [14] , [15] , [16] , [17] , [18] , [19] , [20] , [21] have been constructed to perform various digital logic functions and have demonstrated the great potential of using biological computational circuits [10] , [22] , [23] , [24] to customize cell signalling. However, most of these gene circuits are not modular (that is, they are limited by having to use specific inputs and outputs) or are not insulated from their host chassis (that is, they are limited by having to operate in a specific genetic background to avoid potential cross-talk or at the cost of affecting the host genetic machinery). These limitations prevent their reuse and rapid incorporation into larger biological systems to achieve more complex logic functions. Ideally, a genetic logic device should be modular and orthogonal to their host chassis to facilitate its reuse and reliability in different contexts. Nevertheless, the effort in designing modular and orthogonal genetic devices is largely constrained by the fact that there are only a limited number of orthogonal regulatory components in the current toolbox of gene circuit engineering [25] , such as transcription factor tetR , cI , luxR genes and their regulatory promoters. Hence, a pressing need is to extend this limited parts list, for example, by exploiting and re-engineering the diverse, naturally evolved orthogonal biological control modules in many organisms. Here we constructed a novel modular and orthogonal AND gate in Escherichia coli , using an orthogonal σ 54 -dependent hrpR / hrpS hetero-regulation module from the hrp (hypersensitive response and pathogenicity) system for Type III secretion in Pseudomonas syringae [26] , [27] , [28] . One advantage of the σ 54 -dependent transcription, in contrast to σ 70 , is that it allows very tight control of gene activation, because the RNAP-σ 54 -promoter DNA complex very rarely isomerizes spontaneously to form the transcriptionally competent open complex [29] . The high-order functional forms of the two cooperative activator proteins, HrpR and HrpS [30] , assist the generation of a nonlinear digital-like response of the device. Traditional approaches [31] to gene circuit construction typically build a prototype of the circuit, and then carry out a laborious process of trial-and-error to modify the underlying components, before the desired performance is achieved or use directed evolution [32] , [33] , [34] , [35] , to mutate and then screen out the functional designs. The drawbacks of these approaches are the lack of predictability, and the long time and great effort taken to obtain a functional circuit. In addition, the circuit's behaviour in a different context is unpredictable. To resolve these issues, we took a parts-based engineering approach to construct the AND gate by systematically characterizing a set of candidate components in various contexts and then selecting the appropriate ones and their operational context under the guidance of modelling to assemble the circuit. We show that the behaviours of the assembled logic circuits can be effectively predicted from components that have been characterized in the same abiotic and genetic contexts as required for their final operation. We demonstrate that the resulting AND gate is modular by wiring the inputs to different input promoters and the output to a NOT gate module to produce a combinatorial NAND gate. The logic gates are shown to behave robustly across different cellular contexts. Circuit design and control components characterization The AND gate ( Fig. 1 ; Supplementary Fig. S1 ) comprises two co-activating genes hrpR and hrpS and one σ 54 -dependent hrpL promoter, and can integrate two interchangeable environmental signal inputs to generate one interchangeable output. The output hrpL promoter is activated only when both the co-dependent HrpR and HrpS enhancer-binding proteins are present in a heteromeric complex [30] , with the default hrpL promoter activity close to zero. Because of the requirement of modularity, both the inputs and output of the AND gate were designed to be promoters, allowing the inputs to be wired to any input promoters and the output to be connected to any gene modules downstream to drive various cellular responses. However, it is a non-trivial undertaking to select the right components such as the regulated promoters and RBSs (ribosome binding sites) to drive the AND gate and demonstrate it as functional in a corresponding context. This is not only because many of the components are not well characterized or characterized only in their own specific contexts, but also because of the many factors that affect gene expression in living cells, such as the cell chassis [36] , medium [37] (including carbon source), temperature and component embedded sequence context [38] , [39] like the 5′ untranslated region. Instead of using a routine trial-and-error approach, we decided to characterize each candidate part and sub-module systematically in various contexts (both abiotic and genetic) to provide a reliable choice of the components for engineering a functional device in the corresponding context. 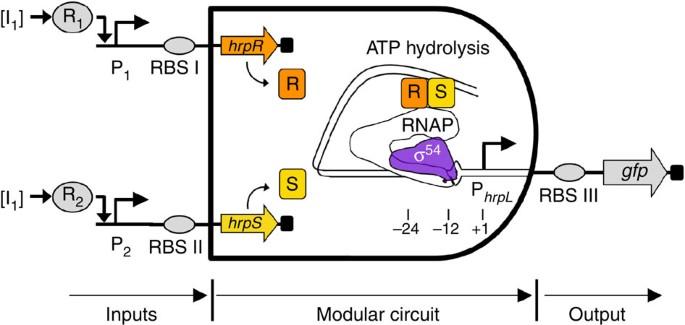Figure 1: A modular and orthogonal genetic AND gate design. The AND gate is designed on the basis of theσ54-dependenthrpR/hrpShetero-regulation module. Two environment-responsive promoters, P1and P2, act as the inputs to drive the transcriptions ofhrpRandhrpS, and respond to the small molecules I1and I2, respectively. The transcription of the outputhrpLpromoter is turned on only when both proteins HrpR and HrpS are present and bind the upstream activator sequence to remodel the closedσ54-RNAP-hrpLtranscription complex to an open one through ATP hydrolysis. The output shown is agfpreporter. The RBS is used for tuning the dynamic range of the device inputs or output. The regulatory promoter inputs andgfpoutput are both interchangeable. The AND gate is orthogonal to theE. coligenetic background and is independent of its normally usedσ70-dependent transcriptional pathway. Figure 1: A modular and orthogonal genetic AND gate design. The AND gate is designed on the basis of the σ 54 -dependent hrpR/hrpS hetero-regulation module. Two environment-responsive promoters, P 1 and P 2 , act as the inputs to drive the transcriptions of hrpR and hrpS , and respond to the small molecules I 1 and I 2 , respectively. The transcription of the output hrpL promoter is turned on only when both proteins HrpR and HrpS are present and bind the upstream activator sequence to remodel the closed σ 54 -RNAP- hrpL transcription complex to an open one through ATP hydrolysis. The output shown is a gfp reporter. The RBS is used for tuning the dynamic range of the device inputs or output. The regulatory promoter inputs and gfp output are both interchangeable. The AND gate is orthogonal to the E. coli genetic background and is independent of its normally used σ 70 -dependent transcriptional pathway. Full size image To verify the integration behaviour of the AND gate, we chose three environment-responsive promoters as the candidate inputs and systematically characterized them—the isopropylthiogalactoside (IPTG) -inducible P lac , the arabinose-inducible P BAD and the quorum signal N -(3-Oxohexanoyl)- L -homoserine lactone (AHL)-inducible P lux ( Supplementary Figs S2 and S3 ). Two cell strains, E. coli MC4100 and E. coli MC1061, which have both P lac and P BAD promoters deleted on their chromosomes, were chosen as the candidate hosts. The chemically well-defined M9 medium was used and supplemented with either glucose (M9-glucose) or glycerol (M9-glycerol) as the carbon source. Six RBSs reported with various translational efficiencies ( Table 1 ) were used to characterize each promoter to find matched promoter/RBS pairs to input into the AND gate. In addition, two temperatures, 30 and 37 °C, were used to evaluate the effect of temperature variations. Table 1 The ribosome binding sites used in this study. Full size table To evaluate the promoter behaviour in different chassis and media, the three regulated promoters were firstly characterized in the two-cell chassis grown in the two media at 30 °C. 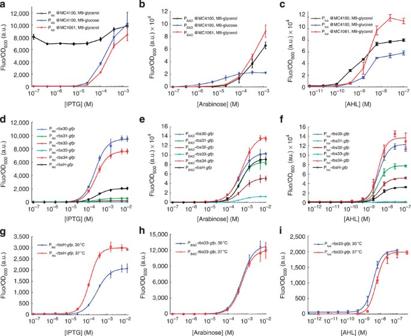Figure 2: Systematic characterization of candidate control elements in various contexts. (a–c) The dose responses of Plac(a), PBAD(b), and Plux(c) promoters to eight increasing induction levels in the two-cell chassis (E. coliMC4100 orE. coliMC1061) in M9-glycerol or M9-glucose media. The samegfpreporter with a strong RBS (rbs30-gfp) was used to measure output fluorescence of the promoter response. (d–f) Dose responses of Plac(d), PBAD, (e), and Plux(f) using 6 versions of RBS under various induction levels (0, 3.9×10−4, 1.6×10−3, 6.3×10−3, 2.5×10−2, 0.1, 0.4, 1.6, 6.4 and 12.8 mM IPTG for Plac; 0, 3.3×10−4, 1.3×10−3, 5.2×10−3, 2.1×10−2, 8.3×10−2, 0.33, 1.3, 5.3 and 10.7 mM arabinose for PBAD; and 0, 1.5×10−3, 6.1×10−3, 2.4×10−2, 9.8×10−2, 3.9×10−1, 1.6, 6.3, 25 and 100 nM AHL for Plux), and the fits (solid lines) to the promoter transfer function. (g–i) The characterized dose responses of Plac(g), PBAD, (h), and Plux(i) under 30 °C and 37 °C, respectively, and the data fits (solid lines). Here rbsH was chosen for Placand rbs33 for PBADand Plux. The inducer concentrations used are the same as ind–f. Ina–i, all data (fluorescence/OD600) were the average of three independent repeats inE. coliMC1061 in M9-glycerol at 30 °C unless otherwise stated. Error bars, s.d. (n=3). a.u., arbitrary units. As Figure 2a shows, P lac is nearly open and does not produce the desired switching characteristics in E. coli MC4100 grown in M9-glycerol, which might be due to an unintended interaction of the P lac with the endogenous genetic background of this host. In E. coli MC4100, grown in M9-glucose ( Fig. 2b ), P BAD is significantly inhibited owing to the catabolite repression effect of glucose (0.01% w/v). P lac is not sensitive to this effect at this level of glucose and is inducible ( Fig. 2a ), while P lux is slightly inhibited ( Fig. 2c ). In E. coli MC1061, grown in M9-glycerol, all the three promoters produced the desired inducible off-on switching characteristics. To identify most-digital-inducible inputs for the AND gate, the conditions ( E. coli MC1061, M9-glycerol, 30 °C) were selected as the standard context for the subsequent characterization work. Figure 2: Systematic characterization of candidate control elements in various contexts. ( a – c ) The dose responses of P lac ( a ), P BAD ( b ), and P lux ( c ) promoters to eight increasing induction levels in the two-cell chassis ( E. coli MC4100 or E. coli MC1061) in M9-glycerol or M9-glucose media. The same gfp reporter with a strong RBS (rbs30- gfp ) was used to measure output fluorescence of the promoter response. ( d – f ) Dose responses of P lac ( d ), P BAD , ( e ), and P lux ( f ) using 6 versions of RBS under various induction levels (0, 3.9×10 −4 , 1.6×10 −3 , 6.3×10 −3 , 2.5×10 −2 , 0.1, 0.4, 1.6, 6.4 and 12.8 mM IPTG for P lac ; 0, 3.3×10 −4 , 1.3×10 −3 , 5.2×10 −3 , 2.1×10 −2 , 8.3×10 −2 , 0.33, 1.3, 5.3 and 10.7 mM arabinose for P BAD ; and 0, 1.5×10 −3 , 6.1×10 −3 , 2.4×10 −2 , 9.8×10 −2 , 3.9×10 −1 , 1.6, 6.3, 25 and 100 nM AHL for P lux ), and the fits (solid lines) to the promoter transfer function. ( g – i ) The characterized dose responses of P lac ( g ), P BAD , ( h ), and P lux ( i ) under 30 °C and 37 °C, respectively, and the data fits (solid lines). Here rbsH was chosen for P lac and rbs33 for P BAD and P lux . The inducer concentrations used are the same as in d – f . In a – i , all data (fluorescence/OD 600 ) were the average of three independent repeats in E. coli MC1061 in M9-glycerol at 30 °C unless otherwise stated. Error bars, s.d. ( n =3). a.u., arbitrary units. Full size image The six RBSs, rbs30-34 plus rbsH, were then used to characterize the three promoters under the selected standard context to seek balanced promoter/RBS pairs. Figure 2d–f show that the maximum response of each promoter varied significantly when using different RBSs. Strikingly, we found that the order of the strengths of the six RBSs across these three promoters varies. This is largely due to the different 5′ untranslated region following each promoter ( Supplementary Fig. S4 ) that can vary the secondary structure and the stability of the transcripts. Clearly, the same part, for example, the RBS, used in different sequence contexts might lead to different quantitative behaviour, as shown in another study [38] . The responses of each promoter, using the six RBSs, become similar after normalization ( Supplementary Fig. S5 ), suggesting the RBS can be used as a linear amplifier to adjust protein expression level at steady state. The effect of temperature variation was investigated by characterizing the promoters at two temperatures 30 and 37 °C, under the otherwise standard culturing condition. Figure 2g–i show that the effect of the shift in temperature on the three promoters is different. For P BAD , a change in temperature from 30 to 37 °C has only a small effect. But P lux becomes leakier at 30 °C than at 37 °C, and P lac has a higher response at 37 °C than at 30 °C. The variations might be due to the different effect of temperature shift on the binding affinities between the transcription factors and their cognate DNA-binding sites of these promoters, suggesting that a change of the abiotic context can have varying impacts on the performance of different parts in an integrated system. The characterization results ( Fig. 2 ), hence, show that the three regulated promoters and six RBSs behave differently in various abiotic (for example, media and temperature) and genetic (for example, chassis and embedded sequence context) contexts. The resulting data ( Fig. 2d–i ) were fitted to a Hill function model for the promoter steady-state input–output response (transfer function) in the form ( Supplementary Methods ): where [ I ] is the concentration of the inducer; K 1 and n 1 are the Hill constant and coefficient, respectively, relating to the promoter–regulator/inducer interaction; k is the maximum expression level due to induction; and α is a constant relating to the basal level of the promoter due to leakage ( Table 2 ). Table 2 The best fits of the characterized promoter responses using different RBSs. Full size table Forward engineering a modular AND gate On the basis of the results of component characterization in various contexts, the AND gate was now systematically designed and constructed by choosing the appropriate parts (input promoters and RBSs) and their relevant context (chassis, media and embedded sequence context). Figure 2d–f show that P lac is much weaker compared with P BAD and P lux promoters. To balance the two driving inputs and avoid potential overexpression, the P lac /rbsH pair input, with a maximum level of around 2,000 a.u. ( Fig. 2d ), was used to drive hrpR , and the P BAD /rbs33 pair, with a maximum level of around 12,000 a.u. ( Fig. 2e ), was used to drive hrpS firstly in the selected standard context ( E. coli MC1061, M9-glycerol, 30 °C). This engineered version of the AND gate exhibited the responses that comply with the function of a Boolean logic AND gate after being measured by fluorometry ( Fig. 3a ). The output is turned on only when both inputs are highly induced, and the response is very sharp in the transition from the off-to-on state and is close to the desired response of a digital logic AND gate. The two-dimensional data were then used to parameterize the normalized transfer function model of the AND gate in the form: This transfer function was derived on the basis of the biochemical interaction underlying the circuit architecture ( Supplementary Methods ). It describes the normalized output of the AND gate as a function of the levels of the two activator proteins ([ R ] for HrpR, [ S ] for HrpS) at steady state. [ G ] max is the maximum activity observed for the output. K R , K S and n R , n S are the Hill constants and coefficients for HrpR and HrpS, respectively. The levels of the two activators were derived from the parameterized transfer functions of the two input promoters ( Table 2 ) with the same RBSs as used in the AND gate. The data fitting with 95% confidence bounds to equation (2) yield: K R =206.1±32.5, K S =3135±374, n R =2.381±0.475 and n S =1.835±0.286 with [ G ] max =7858 a.u. for this assay ( Fig. 3b; Supplementary Fig. S6 ). 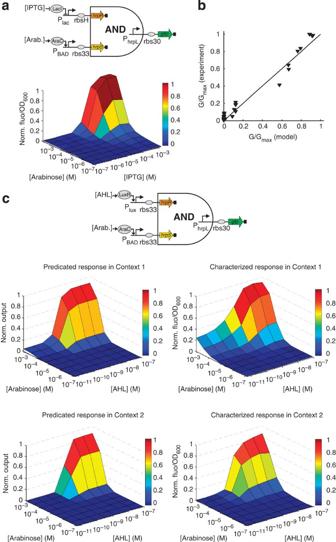Figure 3: Forward engineering a modular AND gate. (a) The AND gate was constructed with Placand PBADpromoters as the two inputs to drive the transcription ofhrpRandhrpS. rbsH and rbs33 are used downstream of Placand PBAD, respectively. The fluorescent response of this device was measured for 72 combinations of input inductions in the standard context as displayed on the bottom. The inducer concentrations used are 0, 3.9×10−4, 1.6×10−3, 6.3×10−3, 2.5×10−2, 0.1, 0.4, 1.6 mM IPTG (left to right) by 0, 3.3×10−4, 1.3×10−3, 5.2×10−3, 2.1×10−2, 8.3×10−2, 0.33, 1.3, 5.3 mM arabinose (bottom to top). (b) The correlation between the AND gate characterized response and predicted response from its fitted transfer function is strong, with Pearson correlation coefficient of 0.9911. Each point represents one experimental data point from the two-dimensional array ina, compared with the model predictedG/Gmaxusing equation (2) and fitted [R] and [S] values from equation (1) for the two characterized promoter inputs. (c) The top is the AND gate with a new configuration, constructed using Pluxand PBADas the two inputs.In silicomodelling predicts the device behaviour in two different contexts (bottom left), that is Context 1 (E. coliMC1061, M9-glycerol, 30 °C) and Context 2 (E. coliMC1061, M9-glycerol, 37 °C). The experimentally characterized responses of the device under these two contexts are on the bottom right. Inducer concentrations used are 0, 2.4×10−2, 9.8×10−2, 3.9×10−1, 1.6, 6.3, 25, 100 nM AHL by 0, 3.3×10−4, 1.3×10−3, 5.2×10−3, 2.1×10−2, 8.3×10−2, 0.33, 1.3 mM arabinose. To be easily compared with the experimental data, the simulations are plotted with the same inducer concentrations as used for characterization. Inaandc, all characterization data are the normalized average of three repeats inE. coliMC1061 in M9-glycerol with variations less than 10% between biological replicates. Figure 3: Forward engineering a modular AND gate. ( a ) The AND gate was constructed with P lac and P BAD promoters as the two inputs to drive the transcription of hrpR and hrpS . rbsH and rbs33 are used downstream of P lac and P BAD , respectively. The fluorescent response of this device was measured for 72 combinations of input inductions in the standard context as displayed on the bottom. The inducer concentrations used are 0, 3.9×10 −4 , 1.6×10 −3 , 6.3×10 −3 , 2.5×10 −2 , 0.1, 0.4, 1.6 mM IPTG (left to right) by 0, 3.3×10 −4 , 1.3×10 −3 , 5.2×10 −3 , 2.1×10 −2 , 8.3×10 −2 , 0.33, 1.3, 5.3 mM arabinose (bottom to top). ( b ) The correlation between the AND gate characterized response and predicted response from its fitted transfer function is strong, with Pearson correlation coefficient of 0.9911. Each point represents one experimental data point from the two-dimensional array in a , compared with the model predicted G / G max using equation (2) and fitted [ R ] and [ S ] values from equation (1) for the two characterized promoter inputs. ( c ) The top is the AND gate with a new configuration, constructed using P lux and P BAD as the two inputs. In silico modelling predicts the device behaviour in two different contexts (bottom left), that is Context 1 ( E. coli MC1061, M9-glycerol, 30 °C) and Context 2 ( E. coli MC1061, M9-glycerol, 37 °C). The experimentally characterized responses of the device under these two contexts are on the bottom right. Inducer concentrations used are 0, 2.4×10 −2 , 9.8×10 −2 , 3.9×10 −1 , 1.6, 6.3, 25, 100 nM AHL by 0, 3.3×10 −4 , 1.3×10 −3 , 5.2×10 −3 , 2.1×10 −2 , 8.3×10 −2 , 0.33, 1.3 mM arabinose. To be easily compared with the experimental data, the simulations are plotted with the same inducer concentrations as used for characterization. In a and c , all characterization data are the normalized average of three repeats in E. coli MC1061 in M9-glycerol with variations less than 10% between biological replicates. Full size image To test the input modularity of the AND gate as well as the validity of its transfer function, we next replaced the P lac input with the AHL-responsive P lux input ( Fig. 3c ). As P lux has been characterized as a strong promoter ( Fig. 2f ), the input of P lux /rbs33 pair (maximum level around 2,000 a.u.) was used to drive the AND gate, close to the input of the P lac /rbsH pair. However, Figure 2i shows that there is greater leakage for P lux at 30 °C than at 37 °C. This behavioural variation of P lux input at these two temperatures might lead to different responses of the assembled AND gate in the two conditions. To evaluate this, we simulated the device behaviour in the two contexts using the component transfer functions that have been parameterized in the corresponding context. The predictions ( Fig. 3c ) show that this AND gate would behave differently in the two contexts, and, especially, a leaky response would appear on the P lux side at the lower temperature context. To confirm the model predictions, the assembled AND gate were experimentally characterized in the two contexts, respectively. Figure 3c shows that the results are consistent with the model predictions ( Supplementary Fig. S6 shows a high correlation coefficient between the two) in that a leaky response on the P lux side was indeed observed for the AND gate at 30 °C. An improved AND gate characteristics of the same device was then obtained in the higher temperature context of 37 °C. These data illustrate that the context in which the circuit performs has a significant impact on its behaviour, and the circuit behaviour can be effectively modelled from the components that have been characterized in the same abiotic and genetic context as required for their final operation. The result also indicates that the inputs of the AND gate are exchangeable and modular. A combinatorial NAND gate To verify the modularity of the AND gate output as well as the forward engineering approach applied, we next connected the AND gate output to a NOT gate module to produce a combinatorial NAND gate. The modular NOT gate was designed on the basis of the cI/P lam repressor module consisting of lambda gene cI and its regulatory P R promoter ( Fig. 4 ). Five versions of the NOT gate, using various RBSs, were constructed and characterized in the selected standard context. 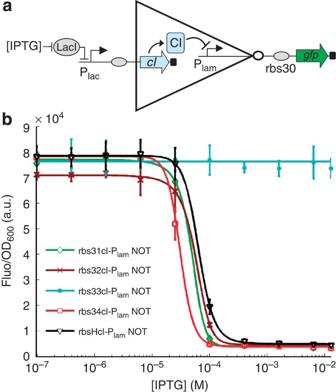Figure 4: A modular NOT gate design and characterization. (a) The design of the modular NOT gate (b) The doses responses of the engineered cI/PlamNOT gate were measured using five versions of RBS under the IPTG-inducible Placpromoter. The inducer concentrations used are 0, 3.9×10−4, 1.6×10−3, 6.3×10−3, 2.5×10−2, 0.1, 0.4, 1.6, 6.4 and 12.8 mM IPTG. The data are the average of three repeats inE. coliMC1061 in M9-glycerol at 30 °C. Solid curves are the data fits to the NOT gate transfer function. Error bars, s.d. (n=3). Figure 4 shows that four of the five versions produced very similar responses and exhibited the required characteristics of a Boolean logic NOT gate—with rapid state transition over a narrow range of inducer concentration, a large dynamic range and a low output level at the off state. The data were fitted to the transfer function of the NOT gate in the form: in which [ R 3 ] is the concentration of the repressor, K 3 and n 3 are the Hill constant and coefficient, k 3 is the maximum expression level without repression and α 3 is a constant relating to the basal level of the regulated promoter ( Supplementary Table S1 ). The levels of the repressor were derived from the parameterized transfer function ( Table 2 ) of the input-inducible promoter with the same RBS as used in the NOT gate. Figure 4: A modular NOT gate design and characterization. ( a ) The design of the modular NOT gate ( b ) The doses responses of the engineered cI/P lam NOT gate were measured using five versions of RBS under the IPTG-inducible P lac promoter. The inducer concentrations used are 0, 3.9×10 −4 , 1.6×10 −3 , 6.3×10 −3 , 2.5×10 −2 , 0.1, 0.4, 1.6, 6.4 and 12.8 mM IPTG. The data are the average of three repeats in E. coli MC1061 in M9-glycerol at 30 °C. Solid curves are the data fits to the NOT gate transfer function. Error bars, s.d. ( n =3). Full size image The composite NAND gate ( Fig. 5a,b ) was then systematically designed on the basis of characterized parts and gate modules. The NAND gate transfer function was derived by integrating the individual transfer functions of the constituent parts (inducible promoters) and modules (AND and NOT gates) in the system ( Supplementary Methods ). We next simulated the device function using parameterized transfer functions of the components that have been characterized in the relevant context. 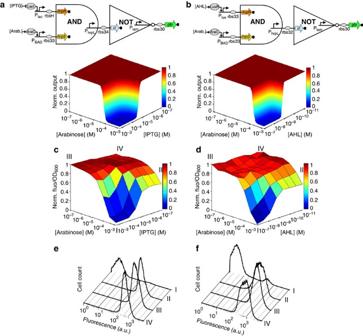Figure 5: Engineering and systematic characterization of a combinatorial NAND gate. (a) The first NAND gate comprises the characterized AND gate module using Placand PBADas inputs and the rbs34-cI/PlamNOT gate module.In silicomodelling predicts the device behaviour based on parameterized transfer functions of the component modules in the standard context. (b) The second NAND gate comprises the AND gate module using Pluxand PBADas inputs and the rbs32-cI/PlamNOT gate module.In silicomodelling predicts the device behaviour based on component parameterized transfer functions at 37 °C under the otherwise standard context. The fitted AND and NOT gate transfer functions at the standard context was used for this simulation and assumed to vary negligibly at 37 °C. (c) Response of the NAND gate as inaunder 64 combinations of input inductions (0, 3.9×10−4, 1.6×10−3, 6.3×10−3, 2.5×10−2, 0.1, 0.4, 1.6 mM IPTG by 0, 3.3×10−4, 1.3×10−3, 5.2×10−3, 2.1×10−2, 8.3×10−2, 0.33, 1.3 mM arabinose) measured by fluorometry in the standard context. (d) Response of the NAND gate as inbfor 64 combinations of input inductions (0, 2.4×10−2, 9.8×10−2, 3.9×10−1, 1.6, 6.3, 25, 100 nM AHL by 0, 3.3×10−4, 1.3×10−3, 5.2×10−3, 2.1×10−2, 8.3×10−2, 0.33, 1.3 mM arabinose) at 37 °C by fluorometry assay. (e) FACS assay of the NAND gate as inaunder four logic combinations of input inductions: (I) 1.3 mM arabinose plus 1.6 mM IPTG, (II) 1.3 mM arabinose, (III) 1.6 mM IPTG, (IV) none. (f) FACS assay of the NAND gate as inbunder four input inductions: (I) 1.3 mM arabinose plus 100 nM AHL, (II) 1.3 mM arabinose, (III) 100 nM AHL, (IV) none. Data incanddare the normalized average of three repeats inE. coliMC1061 in M9-glycerol with variations less than 10% between biological replicates. Figure 5a,b are the predicted characteristics of two versions of the NAND gate with different promoter inputs and configurations. The desired logic NAND function appears in both cases. On the basis of the model predictions, the two NAND gates were constructed by directly assembling the appropriate parts and modules, and were systematically tested in the corresponding context ( Fig. 5c,d ). The two-dimensional input–output responses of the devices comply with the function of a Boolean logic NAND gate. The outputs are in the off state (Point I) only when both inputs are high. The experimental results are close to the model predictions ( Supplementary Fig. S7 ), apart from the slight difference at the corner with low-IPTG and high-arabinose induction on the two-dimensional map (Point II, Fig. 5c ) and, similarly, in Figure 5d , the corner with low-AHL and high-arabinose induction. The minor inhibition at Point II might be due to the slightly leaky expression of HrpR from its control input promoters. Figure 5: Engineering and systematic characterization of a combinatorial NAND gate. ( a ) The first NAND gate comprises the characterized AND gate module using P lac and P BAD as inputs and the rbs34-cI/P lam NOT gate module. In silico modelling predicts the device behaviour based on parameterized transfer functions of the component modules in the standard context. ( b ) The second NAND gate comprises the AND gate module using P lux and P BAD as inputs and the rbs32-cI/P lam NOT gate module. In silico modelling predicts the device behaviour based on component parameterized transfer functions at 37 °C under the otherwise standard context. The fitted AND and NOT gate transfer functions at the standard context was used for this simulation and assumed to vary negligibly at 37 °C. ( c ) Response of the NAND gate as in a under 64 combinations of input inductions (0, 3.9×10 −4 , 1.6×10 −3 , 6.3×10 −3 , 2.5×10 −2 , 0.1, 0.4, 1.6 mM IPTG by 0, 3.3×10 −4 , 1.3×10 −3 , 5.2×10 −3 , 2.1×10 −2 , 8.3×10 −2 , 0.33, 1.3 mM arabinose) measured by fluorometry in the standard context. ( d ) Response of the NAND gate as in b for 64 combinations of input inductions (0, 2.4×10 −2 , 9.8×10 −2 , 3.9×10 −1 , 1.6, 6.3, 25, 100 nM AHL by 0, 3.3×10 −4 , 1.3×10 −3 , 5.2×10 −3 , 2.1×10 −2 , 8.3×10 −2 , 0.33, 1.3 mM arabinose) at 37 °C by fluorometry assay. ( e ) FACS assay of the NAND gate as in a under four logic combinations of input inductions: (I) 1.3 mM arabinose plus 1.6 mM IPTG, (II) 1.3 mM arabinose, (III) 1.6 mM IPTG, (IV) none. ( f ) FACS assay of the NAND gate as in b under four input inductions: (I) 1.3 mM arabinose plus 100 nM AHL, (II) 1.3 mM arabinose, (III) 100 nM AHL, (IV) none. Data in c and d are the normalized average of three repeats in E. coli MC1061 in M9-glycerol with variations less than 10% between biological replicates. Full size image Flow cytometry was used to confirm that the NAND gate functions at individual cellular level. Figure 5e,f show that the entire population is turned off only when both inputs are highly induced (low fluorescent lane I corresponding to Point I in the assay by fluorometery). When either input inducer is not added, the entire population is switched on (high fluorescent lanes II, III and IV). The high fluorescence of a small portion of cells at lane I of the second NAND gate ( Fig. 5f ) might be due to a not fully induced cell population under the induction conditions employed (1.3 mM arabinose plus 100 nM AHL). Particularly, this might be owing to the non-homogeneous input promoter P BAD which shows bimodal activity at subsaturating arabinose conditions in E. coli MC1061 (ref. 40 ) ( Supplementary Fig. S8 ). Circuit chassis compatibility and homogeneity To examine the behaviour of the AND gate in various cell chassis, that is, circuit chassis compatibility, we tested the qualitative responses of the AND gate in seven frequently used E. coli cell strains ( Fig. 6 ). First, the AND gate with P lac and P BAD as the driving inputs was evaluated under four logic input conditions ( Fig. 6a ). The device did not work properly in five out of the seven tested cell chassis— E. coli MC4100, MG1655, DH5α, BW25113 and BL21(DE3). The device behaved well in E. coli MC1061 and TOP10 strains. For most of the non-working chassis, the cells have high output not only with both input inductions but also with only the induction of the P BAD input. These anomalous responses may be due to the interference between the host genetic backgrounds and the P lac promoter input of the device. To confirm this, we then tested the responses of the AND gate using P lux and P BAD as the two inputs under four logic input conditions ( Fig. 6b ). The device now behaved well in all chassis except in E. coli BL21(DE3), a strain with Lon protease gene deleted. The functional improvement of the AND gate among these chassis is, thus, due to the elimination of the potential interference of the input promoter with the host genetic background by using P lux instead of P lac as the first driving input. This is expected because P lux is not endogenous in E. coli and is likely orthogonal to the genetic background of this bacteria, while P lac is an endogenous E. coli promoter and may interact with host background. The levels of the device response on both input inductions vary across the seven tested chassis. Such variation is likely due to the combined effect of the potential interference between the circuit input promoters (P lac and P BAD ) and the host background, and the different growth reductions observed in the experiment for the seven hosts ( Supplementary Tables S2 and S3 ). By combining the two assays, it can be concluded that the AND gate circuit itself is broadly compatible and behaves reliably across most of the tested chassis, but the promoter inputs need to be carefully selected to avoid potential interference with the host genetic background. 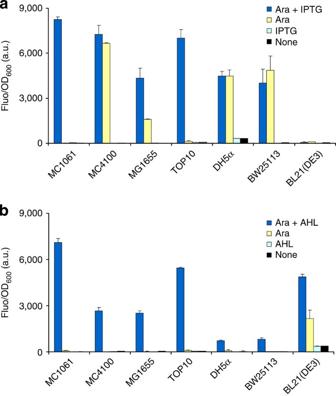Figure 6: Circuit chassis compatibility assays. (a) Qualitative assays of the functionality of the AND gate using Placand PBADas the two inputs in sevenE. colistrains. Four input inductions were studied—1.3 mM arabinose plus 1.6 mM IPTG, 1.3 mM arabinose only, 1.6 mM IPTG only, and no inducers. Cells were grown in M9-glycerol at 30 °C and assayed after 5 h on induction. (b) Qualitative assays of the functionality of the AND gate using Pluxand PBADas the two inputs in sevenE. colistrains. Four input inductions were studied—1.3 mM arabinose plus 100 nM AHL, 1.3 mM arabinose only, 100 nM AHL only, and no inducers. Cells were grown in M9-glycerol at 37 °C and assayed after 5 h on induction. Error bars, s.d. (n=3). Figure 6: Circuit chassis compatibility assays. ( a ) Qualitative assays of the functionality of the AND gate using P lac and P BAD as the two inputs in seven E. coli strains. Four input inductions were studied—1.3 mM arabinose plus 1.6 mM IPTG, 1.3 mM arabinose only, 1.6 mM IPTG only, and no inducers. Cells were grown in M9-glycerol at 30 °C and assayed after 5 h on induction. ( b ) Qualitative assays of the functionality of the AND gate using P lux and P BAD as the two inputs in seven E. coli strains. Four input inductions were studied—1.3 mM arabinose plus 100 nM AHL, 1.3 mM arabinose only, 100 nM AHL only, and no inducers. Cells were grown in M9-glycerol at 37 °C and assayed after 5 h on induction. Error bars, s.d. ( n =3). Full size image We next used flow cytometry to evaluate the population homogeneity of the AND gate circuit, as well as that of the three inducible input promoters ( Supplementary Figs S8 and S9 ). The AND gate was found to be homogeneous in itself. However, the homogeneity of the whole functional device largely relies on the input promoters used, which might not be homogeneous such as the P BAD in E. coli MC1061. The impact of the circuits on the host was evaluated by the growth curves of the cells containing the corresponding constructs. This result ( Supplementary Fig. S10 ) shows that the engineered AND gate placed negligible metabolic load on the host. However, the plasmids used for carrying the circuit constructs can reduce host growth rate, probably due, in a large scale, to the costs of establishing antibiotic resistance for maintaining the plasmids inside the cells. A modular and orthogonal genetic AND gate was constructed in E. coli using a new strictly regulated orthogonal system from P. syringae . The hrpR / hrpS hetero-regulation of the σ 54 -dependent transcription allowed the AND gate to be tightly controlled with a robust near-digital logic behaviour. The device integrated two individual environmental signals through the two transcriptional inputs to generate one output response, accordingly, in the logic AND manner. The AND gate was shown to be modular by exchanging the inputs and output of the circuit while preserving the logic AND function. A modular combinatorial logic NAND gate was generated by directly connecting the AND gate output to a NOT gate module. Because of modularity, the AND and NAND gates can be reconnected to different sensor inputs to integrate multiple environmental and cellular signals [15] , [22] , [41] and thus be applied to identify a specific combinatorial condition, like the cancer microenvironment. The transcription-based AND gate was shown to be robust with functionality in a range of different tested contexts. Moreover, the signal response surfaces of the AND and NAND gates ( Figs 3 and 5 ) show the sigmoid response property for both inputs, largely due to the high cooperativity of the two transcriptional activator proteins. The sigmoidal response filtering property can suppress the analogue noise in biomolecular logic systems and increase signal robustness [42] , [43] , enhancing the error tolerance capability and the scalability of the logic gates. Having a similar role as their electronic counterparts, the engineered AND and NAND gates are the fundamental components in designing biologically based digital systems to control cell signalling and can be easily applied in different contexts, owing to their modularity and orthogonality, to implement human-designed intra- and extra-cellular control functions. Here the genetic logic devices were constructed using a forward engineering approach consisting of quantitative in-context characterization, computational modelling, construction and testing. The results obtained show that both the abiotic and genetic contexts (for example, chassis, medium, temperature and embedded sequence context) in which the parts and modules are placed have a significant impact on their functionality. However, the behaviours of assembled logic circuits were modelled predictably from components when characterized in the same abiotic and genetic context as required for their final operation, implying that, to achieve predictable circuit engineering, individual parts and modules should be in-context characterized to eliminate or reduce any behavioural variations arising from differences in context. The obtained transfer functions of the logic gates implemented here can be used to simulate the behaviour of larger integrated devices or systems [44] when the context in which they are placed is preserved. Alternatively, biological components might be insulated physically [45] and genetically [39] to let them act more stably and predictably in different contexts. Orthogonal parts and modules, such as the AND gate engineered in this study, are important for the compatibility and scalable design of large gene circuits comprising many components. Orthogonality implies that the newly added parts and modules should not cross-talk with those present in the engineered biological systems as well as the host genetic background. The circuit chassis compatibility assays reported here ( Fig. 6 ) indicate that the use of orthogonal and exogenous gene elements for a synthetic circuit in a chassis help to minimize the potential unintended interactions between the circuit and host genetic programmes. Unlike electronic digital circuits, the components in a biological circuit are not connected by wires, and the flow of biological information has to depend on their specific chemical interactions to avoid cross-talk. There is a pressing need to expand the currently limited parts kit of gene circuit engineering. As demonstrated in the construction of the genetic logic gates, the diverse natural building blocks in the myriad of prokaryotic and eukaryotic species provides a rich source from which to engineer orthogonal devices with a variety functions. Plasmid construction Plasmid construction and DNA manipulations were performed following standard molecular biology techniques. The hrpR , hrpS genes and hrpL promoter were synthesized by GENEART following the BioBrick standard ( http://biobricks.org ), that is, eliminating the four restriction sites ( Eco RI, Xba I, Spe I and Pst I) exclusive for this standard by synonymous codon exchange and flanking with prefix and suffix sequences containing the appropriate restriction sites and RBS. The same double terminator BBa_B0015 ( http://partsregistry.org ) was used to terminate gene transcription in all cases. Plasmid pAPT110 (ref. 46 ) (p15A ori, Kan r ) containing the IPTG-inducible P lac was used for P lac promoter characterization and harbouring hrpR ( Xba I/ Kpn I) of the AND gate. Plasmid pBAD18-Cm (ref. 47 ) (pBR322 ori, Cm r ) containing the arabinose-inducible P BAD was used for P BAD promoter characterization and harbouring hrpS ( Xba I/ Kpn I) of the AND gate. pSB3K3 (ref. 48 ) (p15A ori, Kan r ) was used to clone and characterize the synthetic AHL-inducible P lux promoter (BBa_F2620 (ref. 49 )) that was used later to drive hrpR ( Xba I/ Pst I). The hrpL followed by a gfp mut3b reporter construct or a NOT gate module was carried on pSB4A3 (ref. 48 ) (pSC101 ori, Amp r ). The gfpmut3b reporter (BBa_E0840) and NOT gate template (cI/P lam module, BBa_Q04510) was from the Registry of Standard Biological Parts ( http://partsregistry.org ) but introduced with extra restriction site Kpn I at the 3′ end. The NOT gate module was cloned under the IPTG-inducible P lac promoter ( Xba I/ Kpn I) for quantitative characterization. The repressor protein CI in the inverter has been modified with a LVA tail (peptide tag AANDENYALVA) for rapid degradation. The various RBS sequences ( Table 1 ) for each gene construct were introduced by PCR amplification (using PfuTurbo DNA polymerase from Stratagene and an Eppendorf Mastercycler gradient thermal cycler) with primers containing the corresponding RBS and appropriate restriction sites. All constructs ( Supplementary Table S4 ) were verified by DNA sequencing (Eurofins MWG Operon) before their use in target cell strains. Primers ( Supplementary Table S5 ) were synthesized by Eurofins MWG Operon. More information can be found in Supplementary Figure 11 with plasmid maps describing some of the circuit constructs used. Strains and growth conditions Plasmid cloning work was done in E. coli XL1-Blue strain. Characterization work of the circuit constructs were performed in E. coli MC1061 unless otherwise indicated. The extra six E. coli strains used in the circuit chassis compatibility assays are MC4100, MG1655, TOP10, DH5α, BW25113 and BL21(DE3). All characterization experiments were done in M9 minimal media (11.28 g M9 salts/l, 1 mM thiamine hydrochloride, 0.2% (w/v) casamino acids, 2 mM MgSO 4 , 0.1 mM CaCl 2 ), supplemented with appropriate carbon source. Two M9 media with different carbon source were used: M9-glycerol (0.4% (v/v) glycerol) and M9-glucose (0.01% (v/v) glucose). The antibiotic concentrations used were 25 μg ml −1 for kanamycin, 25 μg ml −1 for chloramphenicol and 25 μg ml −1 for ampicillin. Cells inoculated from single colonies on freshly streaked plates were grown overnight in 4 ml M9 in 14 ml Falcon tubes at 37 °C with shaking (200 r.p.m.). Overnight cultures were diluted into pre-warmed M9 media at OD 600 =0.05 for the day cultures, which were induced and grown for 5 h at 30 °C before analysis, unless otherwise indicated. For fluorescence assay by fluorometry, diluted cultures were loaded into a 96-well microplate (Bio-Greiner, chimney black, flat clear bottom) and induced with 5 μl (for single-input induction) or 10 μl (for double-input induction) inducers of varying concentrations to a final volume of 200 μl per well by a multichannel pipette. The microplate was incubated in fluorometer with shaking (200 r.p.m., linear mode) between each cycle of repeat measurements. Assay of gene expression Fluorescence levels of gene expression were assayed by fluorometry at cell population level and by flow cytometry at single-cell level. Cells grown in 96-well plates were monitored and assayed using a BMG POLARstar fluorometer for repeated absorbance (OD 600 ) and fluorescence (485 nm for excitation, 520±10 nm for emission, Gain=1,000) readings (20 min per cycle). Fluorescence-activated cell sorting (FACS) assay were performed using a Becton–Dickinson FACSCalibur flow cytometer with a 488-nm Argon excitation laser and a 530-nm emission filter with 30 nm bandpass. Culture cells were pelleted and resuspended in 0.22 μm filtered PBS. The flow cytometer was tuned with the negative control (GFP-free) to let fluorescence centred within the first decade under log mode and cells scatter at proper location on the scatter graph. Cells were assayed after 5 h growth post-day dilution at low flow rate until 20,000 total events were collected using the BD CellQuest Pro software on a MAC workstation. For flow cytometry assay of the NAND gate, the data were acquired 16 h after induction from cultures inoculated from a single colony containing the circuit. This allows enough cell divisions to completely dilute out the background fluorescent proteins residing in the seed cells because the NAND gate default output is at on state without input inductions. Modelling and data analysis A deterministic approach was used with ODE-based rate equations to model the gene regulation. The transfer functions for the biological modules were derived following a steady-state assumption ( Supplementary Methods ). The nonlinear least square fitting functions (cftool or sftool) in Matlab (MathWorks R2010a) was applied to fit the experimental data to parameterize the transfer function models. The fluorometry data of gene expression were first processed in BMG Omega Data Analysis Software (v1.10) and were analysed in Microsoft Excel 2007 and Matlab after exported. To compensate the effect of evaporation, absorbance readings were calibrated according to the tested evaporation speed (4 μl per hour per well at 30 °C, 8 μl per hour per well at 37 °C). The medium backgrounds of absorbance and fluorescence were determined from blank wells loaded with M9 media and were subtracted from the readings of other wells. The fluorescence/OD 600 (Fluo/OD 600 ) at a specific time for a sample culture was determined after subtracting its triplicate-averaged counterpart of the negative control cultures (GFP-free) at the same time. For population-averaged assay by fluorometry, the fluorescence/OD 600 after 5 h growth post-initial-day dilution and induction was used as the output response of the cells in the steady state when cells were in exponential growth and the steady-state assumption for protein expression is applied ( Supplementary Fig. S3 ). For the NOT and NAND gate assay by fluorometry, the fluorescence values immediately after induction were used as the baseline for the correction of subsequent fluorescence readings. The flow cytometry data were analysed using FlowJo software (v7.2) with an appropriate gate of forward-scattering and side-scattering for all cultures. How to cite this article: Wang, B. et al . Engineering modular and orthogonal genetic logic gates for robust digital-like synthetic biology. Nat. Commun. 2:508 doi: 10.1038/ncomms1516 (2011).